Rab8a interacts directly with PI3Kγ to modulate TLR4-driven PI3K and mTOR signalling Toll-like receptor 4 (TLR4) is activated by bacterial lipopolysaccharide (LPS) to mount innate immune responses. The TLR4-induced release of pro- and anti-inflammatory cytokines generates robust inflammatory responses, which must then be restrained to avoid disease. New mechanisms for the critical regulation of TLR-induced cytokine responses are still emerging. Here we find TLR4 complexes localized in LPS-induced dorsal ruffles on the surface of macrophages. We discover that the small GTPase Rab8a is enriched in these ruffles and recruits phosphatidylinositol 3-kinase (PI3Kγ) as an effector by interacting directly through its Ras-binding domain. Rab8a and PI3Kγ function to regulate Akt signalling generated by surface TLR4. Rab8a and PI3Kγ do not affect TLR4 endocytosis, but instead regulate mammalian target of rapamycin signalling as a mechanism for biasing the cytokine profile to constrain inflammation in innate immunity. Macrophages are key sentinels of the innate immune system, tasked with detecting and responding to pathogens. Accordingly, the macrophage cell surface is armed with various membrane protrusions, is serviced by multiple endocytic and exocytic pathways and has a high rate of plasma membrane turnover to accommodate environmental sampling and pathogen sensing [1] . Members of the Rab family of small GTPases regulate multiple steps of membrane trafficking [2] and, in macrophages, Rabs associated with the cell surface and endocytic pathways are uniquely poised to influence pathogen recognition and internalization [3] , [4] , [5] . Multiple Rabs are involved in the phagocytosis of pathogens [6] , [7] and in the trafficking and secretion of cytokines in pathogen-activated cells [1] . Several Rabs [3] , [4] , [5] have also been implicated in regulating the trafficking of Toll-like receptor 4 (TLR4), a member of the TLR family of pattern recognition receptors that initiate cellular responses to pathogens and danger signals [8] . TLR4 recognizes the lipopolysaccharide (LPS) component of Gram-negative bacteria and activates macrophages to initiate responses including the release of inflammatory cytokines and chemokines, production of reactive oxygen species and modulation of cell survival and proliferation [9] . The spatiotemporal regulation of TLR4 and its signalling from either cell surface or endosomal complexes regulates the net outcome of these responses [10] , [11] , [12] . At the cell surface, LPS-bound TLR4 dimerizes for the phosphoinositide-dependent recruitment of its adaptors, Mal (TIRAP) and MyD88 (ref. 13) [13] , resulting in the activation of transcription factors, such as NFκB and AP-1, for the production of inflammatory cytokines [14] , [15] . Surface activation of TLR4 also invokes the phosphatidylinositol 3-kinase (PI3K)/Akt pathway [16] . Inhibiting PI3Ks biases TLR-induced cytokine responses towards a pro-inflammatory setting. Reports have suggested two mechanisms to explain this effect: the regulation of TLR4 endocytosis [10] and the regulation of downstream TSC/mammalian target of rapamycin (mTOR) signalling [16] . mTOR, a serine/threonine protein kinase, is the catalytic subunit for both the mTORC1 and mTORC2 complexes [17] . Rapamycin targets the mTORC1 complex downstream of Akt, and during TLR4 signalling, it selectively increases the production of pro-inflammatory cytokines [16] . Collectively, these complex signalling pathways regulate the inflammatory response, the programming of which is critical for correctly responding to different pathogens and for delimiting inflammation. Dysregulated or excessive cytokine secretion has serious or even fatal consequences in acute conditions like sepsis, and in chronic inflammatory or autoimmune diseases [18] . Importantly, there are multiple regulatory checkpoints that exert tight control of the TLR4 signalling response; however, the full extent and nature of the mechanisms underlying this control remain unclear. First contact with pathogens such as bacteria is initiated at the cell surface, thus we set out to characterize some of the relevant membrane domains and cellular machinery involved in macrophage activation by LPS. Dorsal ruffles are strikingly upright, and often curved or circular protrusions that accompany pathogen contact and precede macropinocytosis and phagocytosis in activated macrophages [19] , [20] . In other cell types, dorsal ruffles house growth factor receptors and are sites for initiating growth factor-induced signalling [21] , [22] . However, dorsal ruffles have received little previous attention with respect to LPS activation of TLR4 (ref. 19 , 20 ). Screening of Rab GTPases for ruffle localization in macrophages drew our attention to Rab8a, a multi-tasking Rab previously localized to leading edges of the cell surface and endo/exocytic pathways in multiple cell types [23] . Here we show that Rab8a and components of the TLR4 complex are enriched in dorsal ruffles where they contribute to LPS-initiated signalling. By mass spectrometry and biochemical analysis, we identified the p110γ catalytic subunit of PI3K as a new effector for Rab8a and thus present, for the first time, a Rab GTPase that binds directly to a class IB PI3K. Furthermore, we show a function for this complex in innate immune signalling. During TLR4 receptor activation, Rab8a and PI3Kγ are together required to fully activate the Akt/mTOR pathway and bias the cytokine response away from a hyperinflammatory setting by decreasing the production of pro-inflammatory cytokines and increasing the production of anti-inflammatory cytokines. Rab8a and PI3Kγ are presented herein as new regulators of signalling in the TLR4 pathway. TLR4 and Rab8a in dorsal ruffles of activated macrophages In macrophages, peripheral Rac-1 and phosphatidic acid dependent ruffling occurs constitutively [24] and is typically enhanced by growth factors like colony-stimulating factor-1 (ref. 25) [25] . Here we show that LPS also increases dorsal ruffling on macrophages, revealing this as an acute macrophage response to contact with Gram-negative bacteria. F-actin-rich dorsal ruffles protruding from LPS-activated cells are increased twofold over those in untreated cells ( Fig. 1a and Supplementary Fig. 1a ). This mirrors the observation that ruffles do not form after knockdown of TLR4 (ref. 19) [19] . Further examination of ruffles in transfected cells revealed that both Citrine-labelled TLR4 and its cell surface adaptor, Mal (as Cerulean-labelled Mal), are enriched in dorsal ruffles ( Fig. 1b ), denoting these domains as a new location for the pathogen recognition receptor complex of TLR4/Mal/MyD88. Colocalization with Mal places Rab8a in the same ruffles as the TLR4 complex ( Fig. 1c ). Moreover, under these conditions, Rab8a is actively recruited to the ruffles, rather than being present by passive membrane binding alone. This recruitment can be demonstrated by ratiometric imaging, which highlights the dramatic enrichment of full-length Rab8a protein in dorsal ruffles, compared with the charge-dependent membrane binding of the polybasic Rab8a tail ( Fig. 1d and Supplementary Fig. 1b ). As established locales for receptor signalling, dorsal ruffles are enriched in signalling phosphoinositides, PI(3,4,5)P3 and PI(3,4)P2, which can be labelled in live cells with the PH (pleckstrin homology) domain of Akt (GFP-Akt-PH) [26] . Our LPS-activated cells show strong Akt-PH labelling of Rab8a-containing dorsal ruffles, with both molecules enriched two to threefold, compared with their labelling in other plasma membrane domains ( Fig. 1e ). This membrane localization of Rab8a is consistent, even at very low expression levels ( Supplementary Fig. 2 ). Based on Rab8a being enriched in LPS-induced dorsal ruffles, we next investigated a possible role for Rab8a in TLR4 signalling. 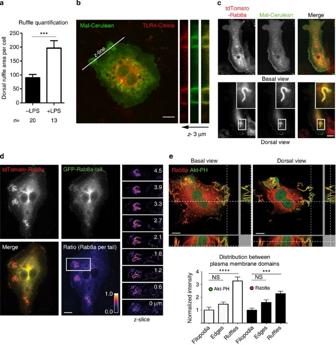Figure 1: Rab8a and TLR4 colocalize in LPS-enhanced dorsal ruffles. (a) Quantification of dorsal ruffling on untreated and LPS-treated RAW 264.7 macrophages. Images of ruffling and parameters for ruffle quantification are shown inSupplementary Fig. 1. The data are analysed by Student’st-test. (n=13–20 per group) ***P<0.001. (b) A single stack image from live, LPS-treated (15 min) RAW 264.7 cells expressing TLR4-Citrine and Mal–Cerulean shows colocalization at peripheral ruffles. Low TLR4-citrine labelling has been enhanced in thez-slice view to visualise cell surface TLR4. Original 16-bit levels (532–18722) enhanced levels (1728–10652). (c) Singlez-stack (0.19 μm slice) image from live cells transfected with Mal–Cerulean and tdTomato-Rab8a. Upper panel shows first three slices from the base of the cell where Rab8a and Mal colocalize at the cell periphery; lower panel shows the top three slices of the cell where there is colocalization in dorsal ruffles. (d) RAW 264.7 cells coexpressing full-length tdTomato-Rab8a and the GFP-tail domain of Rab8a were used to generate ratiometric images to assess Rab8a enrichment at dorsal ruffles. Inset shows 0.6 μmz-slice increments. (e) Singlez-slice shown in basal and dorsal views where td-Tomato Rab8a and GFP-Akt-PH colocalize in ruffles after 15 min of LPS treatment. Quantification of Rab8a and the Akt-PH probe (n=5) in ruffles and other membrane domains was measured by one-way analysis of variance, **P<0.01 and; ****P<0.0001, respectively. Post-test by Dunnett’s multiple comparisons. All images scale bar, 10 μm. Figure 1: Rab8a and TLR4 colocalize in LPS-enhanced dorsal ruffles. ( a ) Quantification of dorsal ruffling on untreated and LPS-treated RAW 264.7 macrophages. Images of ruffling and parameters for ruffle quantification are shown in Supplementary Fig. 1 . The data are analysed by Student’s t -test. ( n =13–20 per group) *** P <0.001. ( b ) A single stack image from live, LPS-treated (15 min) RAW 264.7 cells expressing TLR4-Citrine and Mal–Cerulean shows colocalization at peripheral ruffles. Low TLR4-citrine labelling has been enhanced in the z -slice view to visualise cell surface TLR4. Original 16-bit levels (532–18722) enhanced levels (1728–10652). ( c ) Single z -stack (0.19 μm slice) image from live cells transfected with Mal–Cerulean and tdTomato-Rab8a. Upper panel shows first three slices from the base of the cell where Rab8a and Mal colocalize at the cell periphery; lower panel shows the top three slices of the cell where there is colocalization in dorsal ruffles. ( d ) RAW 264.7 cells coexpressing full-length tdTomato-Rab8a and the GFP-tail domain of Rab8a were used to generate ratiometric images to assess Rab8a enrichment at dorsal ruffles. Inset shows 0.6 μm z -slice increments. ( e ) Single z -slice shown in basal and dorsal views where td-Tomato Rab8a and GFP-Akt-PH colocalize in ruffles after 15 min of LPS treatment. Quantification of Rab8a and the Akt-PH probe ( n =5) in ruffles and other membrane domains was measured by one-way analysis of variance, ** P< 0.01 and; **** P <0.0001, respectively. Post-test by Dunnett’s multiple comparisons. All images scale bar, 10 μm. Full size image Rab8a regulates TLR4 signalling and cytokine secretion To investigate its function, Rab8a was depleted by small hairpin RNA (shRNA) in RAW 264.7 macrophages (to <30% of control levels) and cells were treated with LPS to examine downstream signalling responses ( Fig. 2 ). Rab8a-depleted cells show a modest increase in phosphorylation of the MAPK protein, p38, but no change in ERK1/2 phosphorylation or degradation of the NFκB inhibitory protein, IκB. Notably however, Akt phosphorylation is markedly reduced (by >60% at 30 min) after depletion of Rab8a ( Fig. 2a ). To confirm that the altered Akt response could be attributed to Rab8a, we also examined LPS signalling in cell lines stably overexpressing Rab8a (by approximately three to four fold) and found a ~2.5-fold increase in Akt phosphorylation at 30 and 60 min post LPS ( Supplementary Fig. 3a ). These results serve to implicate Rab8a in TLR4 signalling and suggest that Rab8a is required for maximal PI3K/Akt activation. 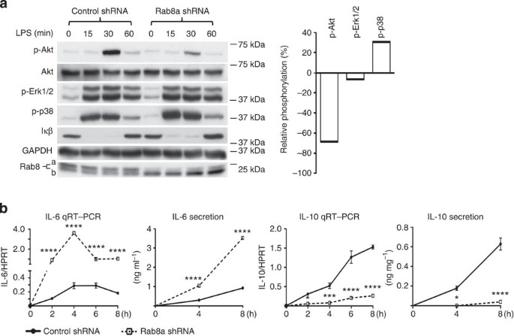Figure 2: Rab8 is required for TLR4-mediated signalling. (a) Representative immunoblot analysis of LPS time course for control (scrambled shRNA) and Rab8a-shRNA stable RAW 264.7 cell lines. Phosphorylation of Akt, ERK1/2 and p38 was analysed at 30 min post LPS by densitometry. All immunoblots were cropped for presentation; full-length blots are provided inSupplementary Fig. 5. (b) Control (scrambled shRNA) and Rab8a-shRNA stable RAW 264.7 cell lines were analysed by quantitative reverse transcriptase PCR (qRT–PCR) for transcriptional response and by enzyme-linked immunosorbent assay for the secretion of the cytokines IL-6 and IL-10. Graphs represent mean±s.e.m. (n=3 each). Time course profiles were analysed by two-way analysis of variance (ANOVA). For qRT–PCR; ****P<0.0001 for both IL-6 and IL-10. For cytokine secretion ****P<0.0001 for IL-6 and ***P<0.001 for IL-10. Two-way ANOVA were analyzed by Sidak’s post-test for multiple comparisons. Figure 2: Rab8 is required for TLR4-mediated signalling. ( a ) Representative immunoblot analysis of LPS time course for control (scrambled shRNA) and Rab8a-shRNA stable RAW 264.7 cell lines. Phosphorylation of Akt, ERK1/2 and p38 was analysed at 30 min post LPS by densitometry. All immunoblots were cropped for presentation; full-length blots are provided in Supplementary Fig. 5 . ( b ) Control (scrambled shRNA) and Rab8a-shRNA stable RAW 264.7 cell lines were analysed by quantitative reverse transcriptase PCR (qRT–PCR) for transcriptional response and by enzyme-linked immunosorbent assay for the secretion of the cytokines IL-6 and IL-10. Graphs represent mean±s.e.m. ( n =3 each). Time course profiles were analysed by two-way analysis of variance (ANOVA). For qRT–PCR; **** P <0.0001 for both IL-6 and IL-10. For cytokine secretion **** P <0.0001 for IL-6 and *** P <0.001 for IL-10. Two-way ANOVA were analyzed by Sidak’s post-test for multiple comparisons. Full size image To test the biological significance of Rab8a depletion, we measured the synthesis and secretion of inflammatory cytokines, which are initiated downstream of LPS-activated TLR4. Over an 8-hour time course, significantly more pro-inflammatory interleukin-6 (IL-6) is produced at both the transcript and secreted levels in Rab8a-depleted cells compared with controls ( Fig. 2b ). Conversely, the Rab8a-depleted cells display decreased synthesis and secretion of the regulatory cytokine, IL-10 ( Fig. 2b ). Thus, Rab8a functions in Akt/PI3K signalling to produce a selective or biased cytokine response to TLR4 activation. This is a wholly new role for Rab8a in TLR4 signalling, and one not readily explained by the known Rab8a effectors [27] . We thus set out to identify the relevant effector(s) or binding partners for Rab8a mediating its involvement in TLR4 signalling. PI3Kγ is a direct binding partner and effector for Rab8a To identify binding partners for Rab8a in macrophages, we performed GST-Rab8a pull-down experiments using LPS-activated cell extracts ( Fig. 3a ). Mass spectrometry analysis revealed a number of known and novel Rab8a-binding partners ( Supplementary Table 1a ). Among them, a prominent but unexpected binding partner emerged as a band at 120 kDa, which was identified convincingly by five independent trypsin-digested peptides, each with 95% confidence ( Fig. 3a,b ), as the p110γ catalytic subunit of PI3K ( Supplementary Tables 1a,b ). Expression of the class 1B PI3Kγ is largely restricted to immune cells where it has been studied in the context of GPCR-dependent neutrophil and T-cell migration [28] , although the highest expression has been reported in myeloid cells, the majority of which are macrophages [29] . To confirm the expression of PI3Kγ in macrophages compared with the other class I PI3Ks (α, β and δ), messenger RNA levels were compared by quantitative reverse transcriptase PCR, and indeed, PI3Kγ is both immune-specific and is the most abundant isoform in macrophages ( Supplementary Fig. 3b ). Traditionally for the class 1B PI3K, the p110γ catalytic subunit interacts with the p87 or p101 regulatory subunits and with the small GTPase Ras for recruitment to GPCRs [30] , [31] . The unexpected binding of PI3Kγ by Rab8a deviates from this model, prompting a more detailed examination to elucidate the nature of this interaction. 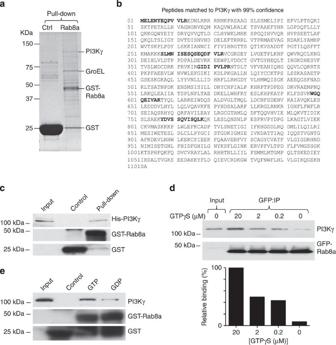Figure 3: Identification of PI3Kγ as a novel effector of Rab8a in macrophages. (a) GST-Rab8a coupled to GSH-Sepharose was used for pull-downs from LPS-activated RAW 264.7 cell extracts. Bound proteins were separated by SDS–PAGE. Excised bands were identified by liquid chromatography/mass spectrometry or mass spectrometry. A major band at 120 kDa, absent from the GST control, was identified as PI3Kγ. (b) The sequence coverage of identified peptides in PI3Kγ. Mass spectrometry analysis identified five trypsin-digested peptides from PI3Kγ with 99% confidence, including many peptides not found in other PI3K isoforms. (c) Coprecipitation of His-PI3Kγ by purified GST-Rab8a. (d) Co-immunoprecipitation of PI3Kγ by GFP-Rab8a in the presence of GTPγS from LPS-treated (15 min) RAW 264.7 cell lysate. Quantification was performed by densitometric analysis of western blots relative to maximal precipitation. (e) Nucleotide exchange of GST-Rab8a with GTP or GDP followed by pull-down of PI3Kγ from RAW 264.7 cell lysate. All immunoblots were cropped for presentation; full-length blots are provided inSupplementary Fig. 5. Figure 3: Identification of PI3Kγ as a novel effector of Rab8a in macrophages. ( a ) GST-Rab8a coupled to GSH-Sepharose was used for pull-downs from LPS-activated RAW 264.7 cell extracts. Bound proteins were separated by SDS–PAGE. Excised bands were identified by liquid chromatography/mass spectrometry or mass spectrometry. A major band at 120 kDa, absent from the GST control, was identified as PI3Kγ. ( b ) The sequence coverage of identified peptides in PI3Kγ. Mass spectrometry analysis identified five trypsin-digested peptides from PI3Kγ with 99% confidence, including many peptides not found in other PI3K isoforms. ( c ) Coprecipitation of His-PI3Kγ by purified GST-Rab8a. ( d ) Co-immunoprecipitation of PI3Kγ by GFP-Rab8a in the presence of GTPγS from LPS-treated (15 min) RAW 264.7 cell lysate. Quantification was performed by densitometric analysis of western blots relative to maximal precipitation. ( e ) Nucleotide exchange of GST-Rab8a with GTP or GDP followed by pull-down of PI3Kγ from RAW 264.7 cell lysate. All immunoblots were cropped for presentation; full-length blots are provided in Supplementary Fig. 5 . Full size image Purified proteins produced in bacterial and insect cells were then used for in vitro- binding assays to confirm that Rab8a binds directly to PI3Kγ ( Fig. 3c ), but not to other class I PI3K isoforms ( Supplementary Fig. 3c ). Furthermore, other Rabs known to function in the TLR4 pathway, such as Rab10 (ref. 3) [3] and 11a [5] , do not co-immunoprecipitate PI3Kγ ( Supplementary Fig. 3d ). This direct interaction is enhanced when Rab8a is in its GTP-bound, active form, as shown by both GTP loading of GST-Rab8a and the co-immunoprecipitation of PI3Kγ by GFP-Rab8a in the presence of increasing concentrations of a non-hydrolysable GTP analogue, GTPγS ( Fig. 3d,e ). These characteristics are consistent with PI3Kγ interacting with GTP-Rab8a as a new class of Rab effector. The recruitment of PI3Kγ to membranes is sufficient to initiate its kinase activity, unlike the other class IA PI3K isoforms [32] . In other signalling pathways, this recruitment is mediated by Ras binding directly to the Ras-binding domain (RBD) of PI3Kγ [30] . To test whether the RBD is similarly responsible for Rab8a binding, we performed pull-down experiments using the isolated recombinant RBD from PI3Kγ. The RBD could successfully substitute for full-length protein under the pull-down conditions, confirming that it is necessary and sufficient for binding to Rab8a ( Fig. 4a ). We then utilized the known crystal structures of GTP-bound Rab8a [33] and the co-crystal structure of PI3Kγ with Ras [34] to produce a homology model of Rab8a/PI3Kγ ( Fig. 4b ). This model shows a viable alignment of the PI3Kγ RBD with the effector-binding domain of Rab8a and predicts the critical binding residues on both sides of the interacting surface. Mutation of either F221 or T232 in the RBD or the I41 residues in the effector-binding domain of Rab8a is sufficient to reduce interaction of the two proteins in pull-down experiments ( Fig. 4c ). These results provide detailed evidence of a direct interaction between Rab8a and PI3Kγ. Rab8a binds to the same RBD as Ras, and moreover, uses the same critical residues in the RBD [34] for its interaction with PI3Kγ. PI3Kγ normally binds to Ras during its recruitment to activated receptor (GPRC or RTK) complexes. Seeking evidence for such a receptor interaction with TLR4 revealed that PI3Kγ does not co-immunoprecipitate with TLR4 ( Supplementary Fig. 3e ). Taken together, the substitution of Ras with Rab8a and the recruitment of PI3Kγ independently of TLR4 imply a novel mode for recruitment of PI3Kγ in the TLR4 pathway. 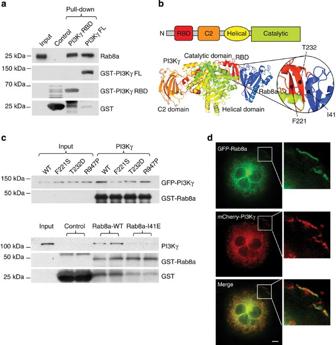Figure 4: Characterization of Rab8a and PI3Kγ interaction. (a) Bacterially expressed GST-PI3Kγ RBD (amino acids 1–356) and insect cell-expressed full-length GST-PI3Kγ were used to pull down Rab8a from RAW 264.7 cell lysates. (b) PI3Kγ domain structure and homology model of the Rab8a/PI3Kγ complex. The homology model was generated using the crystal structure of GTP-bound Rab8a (PDB:3QBT) and the co-crystal of PI3Kγ and Ras (PDB:1HE8). (c) Pairwise GST pull-down experiment using either the mutant forms of PI3Kγ with wild-type Rab8a or mutated Rab8a with wild-type PI3Kγ. All Rab8 fusion proteins were GTP-loaded. The kinase-inactive mutant (R947P) was used as a negative control. (d) LPS-treated (15 min) RAW 264.7 macrophages cotransfected with GFP-Rab8a and mCherry-PI3Kγ show colocalization in ruffles. Scale bar, 10 μm. All immunoblots were cropped for presentation; full-length blots are provided inSupplementary Fig. 5. Figure 4: Characterization of Rab8a and PI3Kγ interaction. ( a ) Bacterially expressed GST-PI3Kγ RBD (amino acids 1–356) and insect cell-expressed full-length GST-PI3Kγ were used to pull down Rab8a from RAW 264.7 cell lysates. ( b ) PI3Kγ domain structure and homology model of the Rab8a/PI3Kγ complex. The homology model was generated using the crystal structure of GTP-bound Rab8a (PDB:3QBT) and the co-crystal of PI3Kγ and Ras (PDB:1HE8). ( c ) Pairwise GST pull-down experiment using either the mutant forms of PI3Kγ with wild-type Rab8a or mutated Rab8a with wild-type PI3Kγ. All Rab8 fusion proteins were GTP-loaded. The kinase-inactive mutant (R947P) was used as a negative control. ( d ) LPS-treated (15 min) RAW 264.7 macrophages cotransfected with GFP-Rab8a and mCherry-PI3Kγ show colocalization in ruffles. Scale bar, 10 μm. All immunoblots were cropped for presentation; full-length blots are provided in Supplementary Fig. 5 . Full size image We then sought to determine the membrane localization of Rab8a and PI3Kγ. Cotransfected macrophages show diffuse cytoplasmic labelling of mCherry-PI3Kγ, typical of PI3K isoforms. In LPS-activated cells, PI3Kγ is recruited to macrophage ruffles where it colocalizes with GFP-Rab8a ( Fig. 4d ). Like all class I PI3K isoforms, PI3Kγ converts PI(4,5)P2 to PI(3,4,5)P3, a function that is in keeping with the phosphoinositide environment of the Rab8-positive ruffles (shown in Fig. 1e ). Thus we introduce the class IB PI3Kγ as a novel effector for GTP-Rab8a on ruffle membranes. Next, we further examined this contention by testing whether PI3Kγ, like Rab8a, functions in TLR4 signalling. PI3Kγ depletion effects on TLR4 signalling and inflammation As the first of three approaches to explore PI3Kγ function, we used independent small interfering RNAs targeting PI3Kγ ( Fig. 5a ). For all small interfering RNAs, there was a decrease in the phosphorylation of Akt after LPS treatment that correlated with the depletion level of PI3Kγ ( Fig. 5a ). As a second approach, macrophages were treated with a PI3Kγ isoform-specific inhibitor, AS605240 (ref. 35) [35] , resulting in reduced phosphorylation of Akt in a dose-dependent manner ( Fig. 5b ). As PI3Kγ inhibitors can have off-target effects at higher concentrations, we also used genetic ablation of PI3Kγ in knockout mice to assess its function. Targeted knockout of the p110γ subunit (PI3Kγ −/− ) in the C57BL/6 mouse background does not affect the expression of other p110 isoforms (α, β and δ) [28] . Primary bone marrow-derived macrophages (BMMs) from PI3Kγ −/− and wild-type mice were challenged with LPS, resulting in >50% decreased phosphorylation of Akt in PI3Kγ-null cells ( Fig. 5c ). Taken together, these findings indicate that loss of PI3Kγ in LPS-treated macrophages significantly reduces Akt signalling. This effect mimics the knockdown of Rab8a (see Fig. 2a,b ) and is consistent with the notion that PI3Kγ acts as the Rab8a effector during TLR4 signalling. We therefore deduce that the physiological roles of both Rab8a and PI3Kγ are to augment TLR4-mediated PI3K/Akt signalling. 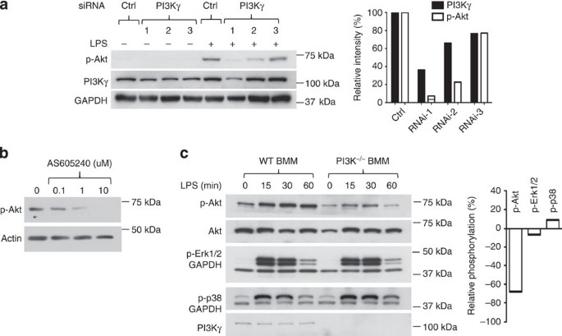Figure 5: PI3Kγ regulates TLR4-mediated signalling in macrophages. (a) RAW 264.7 macrophages treated with either control (non-targeting), or one of three independent PI3Kγ-targeting small interfering RNAs were incubated with LPS for 30 min. Quantification of western blots was performed using densitometry. (b) RAW 264.7 cells were treated for 30 min with either vehicle (DMSO), 0.1, 1 or 10 μM of AS605240 before addition of LPS for 30 min. Cell extracts were analysed for Akt phosphorylation. (c) BMMs derived from wild-type (WT) and PI3Kγ−/−animals were subjected to a 60-min time course of LPS. Cell extracts were analysed for Akt, ERK1/2 and p38 phosphorylation. Quantification of phosphorylation is at the 30-min time point only and the gel is representative (n=3 each). All immunoblots were cropped for presentation; full-length blots are provided inSupplementary Fig. 6. Figure 5: PI3Kγ regulates TLR4-mediated signalling in macrophages. ( a ) RAW 264.7 macrophages treated with either control (non-targeting), or one of three independent PI3Kγ-targeting small interfering RNAs were incubated with LPS for 30 min. Quantification of western blots was performed using densitometry. ( b ) RAW 264.7 cells were treated for 30 min with either vehicle (DMSO), 0.1, 1 or 10 μM of AS605240 before addition of LPS for 30 min. Cell extracts were analysed for Akt phosphorylation. ( c ) BMMs derived from wild-type (WT) and PI3Kγ −/− animals were subjected to a 60-min time course of LPS. Cell extracts were analysed for Akt, ERK1/2 and p38 phosphorylation. Quantification of phosphorylation is at the 30-min time point only and the gel is representative ( n =3 each). All immunoblots were cropped for presentation; full-length blots are provided in Supplementary Fig. 6 . Full size image We also examined the downstream cytokine responses to LPS in PI3Kγ −/− BMMs, where production of pro-inflammatory cytokines, IL-6 and IL-12p40, is significantly enhanced in response to LPS, compared with BMMs from control animals ( Fig. 6a,b ). In contrast, the synthesis and release of IL-10 and the anti-viral type I interferon, IFN-β, are significantly suppressed in PI3Kγ −/− BMMs. Hence, PI3Kγ affects not only signalling, but also the innate immune responses activated by TLR4 in macrophages. In keeping with the signalling profiles and with the role of Rab8a, PI3Kγ serves to bias the inflammatory response by constraining the production of pro-inflammatory cytokines. 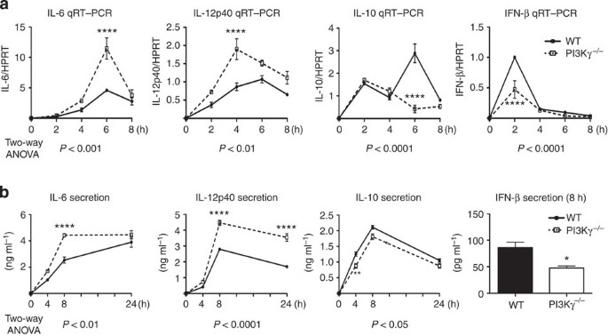Figure 6: PI3Kγ attenuates the inflammatory response. (a) Quantitative reverse transcriptase PCR time course after LPS treatment in WT and PI3Kγ−/−BMMs. Data points are the mean±s.e.m. (n=3) of cytokine profiles and were compared by two-way analysis of variance (ANOVA). (b) Cytokines secreted into the BMM medium were measured by enzyme-linked immunosorbent assay, post-LPS treatment, with the exception of IFN-β, which was measured at 24 h. Each data point is the mean±s.e.m. (n=3 with three replicates). Significance was measured by two-way ANOVA with Sidak’s post-test for multiple comparisons (**P<0.01, ****P<0.0001). IFN-β was measured by Student’st-test. Figure 6: PI3Kγ attenuates the inflammatory response. ( a ) Quantitative reverse transcriptase PCR time course after LPS treatment in WT and PI3Kγ −/− BMMs. Data points are the mean±s.e.m. ( n =3) of cytokine profiles and were compared by two-way analysis of variance (ANOVA). ( b ) Cytokines secreted into the BMM medium were measured by enzyme-linked immunosorbent assay, post-LPS treatment, with the exception of IFN-β, which was measured at 24 h. Each data point is the mean±s.e.m. ( n =3 with three replicates). Significance was measured by two-way ANOVA with Sidak’s post-test for multiple comparisons (** P< 0.01, **** P <0.0001). IFN-β was measured by Student’s t -test. Full size image PI3Kγ does not regulate endocytosis of TLR4 The internalization of TLR4 (ref. 12) [12] by effectively removing it from the surface adaptors, Mal and MyD88, is one possible mechanism for limiting pro-inflammatory signalling [10] . Since class I PI3Ks are commonly involved in endocytic pathways [36] and Rabs are also common endocytic regulators [37] , a plausible mechanism for the actions of Rab8a/PI3Kγ would ostensibly be to regulate the endocytosis of TLR4. However, testing of known endocytic pathways in PI3Kγ −/− BMMs revealed no requirement for PI3Kγ in directly regulating FcγR-mediated phagocytosis, clathrin-mediated transferrin receptor endocytosis or dextran-labelled macropinocytosis ( Supplementary Fig. 4a–c ). Thus, common endocytic pathways in PI3Kγ-null mice appear to operate efficiently. The internalization of TLR4 itself was then measured by surface immunolabelling and flow cytometry over a time course of LPS activation. 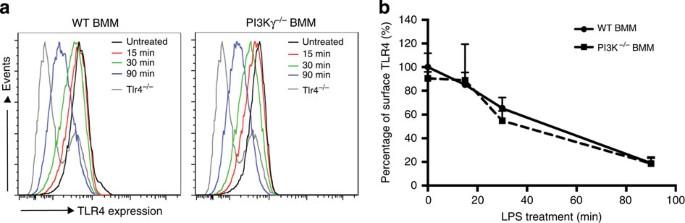Figure 7: Endocytosis of surface TLR4 is not PI3Kγ-dependent. (a) Untreated or LPS-treated (100 ng ml−1for the times indicated) WT and PI3Kγ−/−BMMs were used to examine surface levels of endogenous TLR4 by immunostaining and flow cytometry. (b) Quantification of TLR4 internalization over time. The percentage of surface TLR4 was calculated by the mean fluorescent intensity of TLR4 receptor staining at each time point over MFI of untreated cells (n=3 with three replicates). TLR4 is successfully internalized in PI3Kγ −/− BMMs at the same rate as in control cells ( Fig 7a,b ). Hence, PI3Kγ is not required to regulate the endocytosis of TLR4 in this context. Figure 7: Endocytosis of surface TLR4 is not PI3Kγ-dependent. ( a ) Untreated or LPS-treated (100 ng ml −1 for the times indicated) WT and PI3Kγ −/− BMMs were used to examine surface levels of endogenous TLR4 by immunostaining and flow cytometry. ( b ) Quantification of TLR4 internalization over time. The percentage of surface TLR4 was calculated by the mean fluorescent intensity of TLR4 receptor staining at each time point over MFI of untreated cells ( n =3 with three replicates). Full size image PI3Kγ mediates cytokine biasing through mTOR A second mechanistic explanation for the cytokine bias observed in Rab8a- and PI3Kγ-depleted cells involves the mTORC1 complex, which acts downstream of PI3K in TLR4 pathways. Within this complex, the serine/threonine protein kinase mTOR has been implicated in the transcriptional and post-translational regulation of cytokine production and biasing [38] . In our wild-type BMMs, inhibition of mTORC1 with rapamycin effectively enhances the production of pro-inflammatory cytokines, IL-6 and IL-12p40, while decreasing the levels of IL-10 ( Fig. 8a ). This is roundly consistent with the effects of Rab8a and PI3Kγ on cytokine outputs in our experiments, and with findings relating to mTOR function in the literature [16] , [39] . To investigate if PI3Kγ regulates mTOR downstream of TLR4, we analysed the phosphorylation of Akt and mTOR in LPS-treated wild-type and PI3Kγ −/− BMMs ( Fig. 8b ). Quantification revealed a significant reduction in both Akt and mTOR phosphorylation in the absence of PI3Kγ ( Fig. 8b ). To investigate the significance of the decreased mTOR phosphorylation, we tested two canonical mTORC1 substrates, 4E-BP1 and p70S6K, known targets during LPS stimulation [16] . In PI3Kγ −/− cells after LPS treatment, the phosphorylation of p70S6K was reduced to below detectable levels, while 4E-BP1 phosphorylation was reduced for the higher molecular weight isoform. Together, these results confirm a defect in the PI3K/Akt/mTOR pathway ( Fig. 8c ). Thus, PI3Kγ is required for efficient activation of mTOR in response to pathogen recognition by TLR4. Taken together, our data suggest a new role for PI3Kγ during TLR4 signalling and one that is independent of receptor endocytosis. The recruitment of Rab8a and PI3Kγ during TLR4 activation functions to enhance the mTOR signalling pathway, effectively polarizing the cytokine response and limiting inflammation. 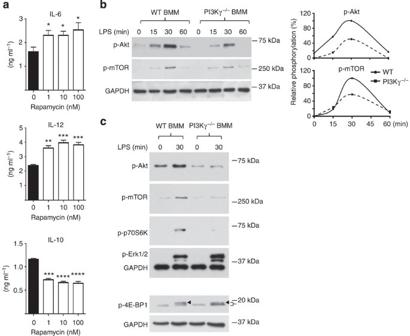Figure 8: PI3Kγ regulation of mTOR during TLR4 signalling. (a) Cytokines secreted into the medium of untreated and mTOR inhibitor (rapamycin)-treated BMMs were measured by enzyme-linked immunosorbent assay, post-LPS treatment at 8 h. Data points are the mean±s.e.m. (n=5 with three replicates). Significance was measured Student’st-test (*P<0.05, **P<0.01, ***P<0.001, ****P<0.0001) (b) BMMs derived from WT and PI3Kγ−/−animals were subjected to a 60-min time course of LPS. Cell extracts were analysed for Akt and mTOR phosphorylation. Densitometric quantification of phosphorylation is at the 30-min time point only and the gel is representative (n=3 each). (c) BMMs derived from WT and PI3Kγ−/−animals were treated with LPS (30 min) and cell extracts were analysed for phosphorylation of the mTOR substrates, p70S6K and 4E-BP1. Arrow heads indicate the hyperphosphorylated form of 4E-BP1, which has a mobility shift. All immunoblots were cropped for presentation; full-length blots are provided inSupplementary Fig. 6. Figure 8: PI3Kγ regulation of mTOR during TLR4 signalling. ( a ) Cytokines secreted into the medium of untreated and mTOR inhibitor (rapamycin)-treated BMMs were measured by enzyme-linked immunosorbent assay, post-LPS treatment at 8 h. Data points are the mean±s.e.m. ( n =5 with three replicates). Significance was measured Student’s t -test (* P< 0.05, ** P< 0.01, *** P< 0.001, **** P <0.0001) ( b ) BMMs derived from WT and PI3Kγ −/− animals were subjected to a 60-min time course of LPS. Cell extracts were analysed for Akt and mTOR phosphorylation. Densitometric quantification of phosphorylation is at the 30-min time point only and the gel is representative ( n =3 each). ( c ) BMMs derived from WT and PI3Kγ −/− animals were treated with LPS (30 min) and cell extracts were analysed for phosphorylation of the mTOR substrates, p70S6K and 4E-BP1. Arrow heads indicate the hyperphosphorylated form of 4E-BP1, which has a mobility shift. All immunoblots were cropped for presentation; full-length blots are provided in Supplementary Fig. 6 . Full size image In this study, we describe a new regulatory unit consisting of Rab8a with PI3Kγ as its effector. In this context, Rab8a plays a new role in signalling with novel PI3Kγ function in the TLR4 pathway. This additional role for PI3Kγ extends its reach beyond known GPCRs and RTKs. In macrophages exposed to LPS, Rab8a and PI3Kγ are recruited to dorsal ruffles along with components of the TLR4/Mal/MyD88 complex. Rab8a and PI3Kγ are two newly introduced partners that are required for effective Akt/mTOR signalling during TLR4 activation. PI3Kγ serves to enhance mTOR phosphorylation and signalling via this arm of the TLR4 response, whereby downstream proteins can both constrain inflammatory responses by curtailing production of pro-inflammatory cytokines and bias the response in favour of regulatory or anti-inflammatory cytokines [38] . Our findings thus reveal the Rab8a/PI3Kγ complex as an important and additional mechanism for controlling PI3K signalling in inflammation. Rab8a is a ubiquitous Rab, functioning in multiple recycling pathways through a variety of effectors [27] , [40] , [41] . The Rab8a localization we show in activated macrophages is broadly commensurate with its previous localization on cell surfaces, at leading edges and on membrane vesicles and tubules moving to and from the surface [23] , [40] . Within this distribution, we show a specific and dramatic recruitment of Rab8a to dorsal ruffles on the surface of LPS-activated macrophages, along with components of the surface TLR4 complex. Our study serves to highlight macrophage dorsal ruffles as a previously unheralded site for clustering of the TLR4 receptor and associated molecules. The features we show, namely the recruitment of PI3Kγ, generation of the signalling phosphoinositide PI(3,4,5)P3 and subsequent activation of Akt, denote these dorsal ruffles as a functional site for TLR4 signalling. Rab8a enrichment in the ruffles is striking and reflects the clustering of Rabs at functional membrane domains, mostly at the behest of their guanine nucleotide exchange factors and effectors. The identity of such Rab8a recruitment factors in this locale is not yet known, although the GTPase Arf6 is a candidate player due to its roles in ruffle formation [42] , its deactivation of Rab8a in epithelial cells [43] and a proposed role in TLR4 activation in macrophages [13] . While Rab8a regulates signalling from the surface TLR4 complex, additional Rabs influence TLR4 at other points along the endocytic and recycling pathways via more traditional trafficking mechanisms. Rab11a regulates recycling endosome-mediated delivery of TLR4 to phagosomes, an alternative site proposed for LPS activation of TLR4 wherein TLR4 signals via the TRIF/TRAM adaptors to produce IFN-β 5 . Of note is the fact that phagosomes can be generated from dorsal ruffles, suggesting perhaps another route for spatiotemporal regulation of TLR4. Also, Rab10 (ref. 3) [3] and Rab7 (ref. 4) [4] function in recycling of TLR4 to the surface and for degradation, respectively; however, Rab effectors relevant to TLR4 at all of these other steps remain undefined. We now recast Rab8a with a new effector and a very different role through its direct involvement in PI3K signalling in the TLR4 pathway. PI3Kγ was revealed herein as an unexpected binding partner for Rab8a and the first instance of class 1B PI3Ks directly interacting with a Rab. Rab5 was previously implicated as an effector for class IA PI3Kβ [44] , although the nature of this interaction was not characterized. At a molecular level, the PI3K catalytic subunit p110γ is traditionally recruited by binding directly to Ras, along with a class IB regulatory subunit, and the Gβγ subunit of an activated GPCR complex [45] . We now confirm that Rab8a and PI3Kγ bind directly to each other, using homology modelling and mutagenesis of critical residues. Rab8a binds to two residues in the RBD of PI3Kγ that are critical and necessary for Ras binding to PI3Kγ [34] . Recently, Rho family GTPases, Rac1 and CDC42, but not Ras, were also shown to directly interact with class IA PI3Kβ through the kinase’s RBD [46] . Our findings now show that the PI3K RBD also supports interactions with a Rab GTPase, in addition to Ras and Rho family GTPases [46] . These G protein families thus offer a variety of modalities for the recruitment and regulation of PI3Ks in signalling pathways. In the context of LPS signalling, it remains unclear precisely how PI3Kγ is recruited and activated by TLR4, particularly because PI3Kγ does not bind directly to TLR4. Our findings suggest that Rab8a provides a parallel means of recruiting a PI3K to augment LPS signalling, with Rab8a/PI3Kγ acting as an auxiliary unit in its own right or in the context of another receptor. Such crosstalk for amplifying PI3K-mediated signalling has precedents, including the Fc?RI receptor in mast cells, where this receptor has no direct link to GPCRs, yet degranulation is dependent on PI3Kγ [47] . Indeed, a seminal study of tumour-associated macrophages expanded the field of PI3Kγ’s influence by showing that it regulates signalling not only from GPCRs, but also from RTKs and the TLR/IL1 receptor [29] . In the complex ligand environment of tumour inflammation, the loss of PI3Kγ was found to limit tumour progression [29] , in line with the current interest in PI3Kγ inhibitors for treating cancer. By adding the pathogen recognition receptor, TLR4, to the classes of receptors employing PI3Kγ, we raise questions for the future about even more receptors that may activate Rab8a/PI3Kγ, including other members of the TLR family and their arrays of pathogen-derived ligands. Further studies are also needed to establish whether Rab8a, rather than Ras, is involved in recruiting PI3Kγ to other receptor families. Previous studies have focused on TLR4 internalization as a mechanism by which macrophages can terminate the production of pro-inflammatory cytokines [10] , [11] , [12] . The class IA PI3Kδ is recruited to the TLR4 complex, where it reportedly regulates internalization of the receptor by an unknown pathway [10] . This results in a switch from cell surface MyD88/Mal signalling, which generates pro-inflammatory cytokines, to the endosomal adaptors TRIF/TRAM, which induce production of type I interferons [10] . We saw no general effects on endocytosis or the internalization of TLR4 itself after loss of PI3Kγ. Therefore, Rab8a/PI3Kγ operates via another mechanism to control TLR4 signalling and cytokine production. The effects we demonstrate here for PI3Kγ are similar to those reported for PI3Kδ in enhancing Akt signalling and in limiting pro-inflammatory cytokines. Therefore, it is likely that both PI3Ks act in concert to augment the same effect, possibly reflecting the need for multiple mechanisms to stimulate and fine-tune the production of inflammatory cytokines. Mechanistically, we found that Rab8a and PI3Kγ exert their control over cytokine production by signalling through the multi-functional serine/threonine protein kinase mTOR, which acts as a hub downstream of TLR4 to strategically bias cytokine responses [48] . In this context, mTOR signalling inhibits the function of NFκB and the transcription of pro-inflammatory cytokines, IL-6 and IL-12p40, while enhancing the function of STAT3 and the transcription of an anti-inflammatory or regulatory cytokine, IL-10 (refs 16 , 49 ). The importance of mTOR in this regulatory role emerged with a recent study showing that the intracellular pathogen Legionella pneumophila subverts the immune response with bacterial effectors that target mTOR to disengage its cytokine biasing role [39] . The regulation of mTOR downstream of TLR4 by PI3Kγ results in the polarized inflammatory response towards an anti-inflammatory setting. This effect has been demonstrated elsewhere, through the pharmacological inhibition of mTORC1 with rapamycin and by the genetic perturbation of TSC2—another kinase in the pathway [16] . Our findings represent the first example of mTOR regulation by a Rab GTPase through PI3Kγ. Given that mTOR controls many cellular functions, Rab8a and PI3Kγ may have broader physiological effects beyond cytokine production. PI3Kγ has become an attractive drug target in cancer and other diseases [50] . PI3Kγ −/− mice show reduced inflammation in a number of disease models, including diabetes [51] and cardiovascular disease [52] , primarily related to roles for this kinase in GPCR-dependent cell migration of immune cells and activation of the respiratory burst [28] . On this basis, PI3Kγ inhibitors are also viewed as potential anti-inflammatory drugs [47] . However, at least in the context of bacterial infection, our preliminary results suggest that PI3Kγ inhibition might acutely skew signalling towards pro-inflammatory cytokines, enhancing bactericidal responses, but exacerbating inflammation. Further studies are now needed to dissect the role of PI3Kγ and the clinical consequences of its inhibition over the course of bacterial infection and in disease. As a pharmacologically tractable target operating at a critical point to regulate cytokine outputs from TLR4 activation, understanding how PI3Kγ influences infection and inflammatory disease is vital. Antibodies and reagents Primary antibodies recognizing PI3Kα, β, γ, δ (sampler kit-9655), phospho-mTOR, phospho-4E-BP, phospho-p70 S6 kinase (sampler kit-9862), Akt (9272), phospho-Akt (Ser 473 ) (4962), phospho-p38 MAPK (Thr 180 /Tyr 182 ) (4511), IκBα (9242), phospho-ERK1/2 (4370) were purchased from Cell Signaling Technology (Beverly, MA, USA). Mouse anti-Rab8 (610845) was purchased from BD Transduction Laboratories (Lexington, KY, USA). GST antibody (71-7500) was purchased from Invitrogen, Sydney, Australia. Anti-TLR4 for western blotting was from Abcam (ab22048). For fluorescent-activated cell sorting (FACS) analysis, the anti-TLR4 SA15-21 clone was biotinylated using the EZ-Link Micro Sulfo-NHS-LC-Biotinylation Kit (Thermo Scientific, CA, USA). Streptavidin–APC (Biolegend, CA, USA) was used to detect biotinylated anti-TLR4. Mouse anti-glyceraldehyde-3-phosphate dehydrogenase (2275-PC-1) was purchased from Trevigen (Gaithersburg, MD, USA). Alexa Fluor 488/594- (A21208) and 647- (A31573) conjugated secondary antibodies, Alexa Fluor 488- and 647-dextran and wheat germ agglutinin (WGA)-Texas Red were purchased from Molecular Probes (Invitrogen, OR, USA). Horseradish peroxidase-conjugated goat anti-mouse and rabbit antibodies (81–6520) were obtained from Zymed (San Francisco, CA, USA). Bacterial lipopolysaccharide (LPS), purified from Salmonella enterica serotype Minnesota Re 595, was purchased from Sigma-Aldrich (Castle Hill, NSW, Australia). AS605240 (IC 50 =0.008 μM) was purchased from Sigma-Aldrich and IC87114 (IC 50 =0.07 μM) was from Scientifix, Australia. For phagocytosis, human IgG (Invitrogen) was conjugated to 3 μm latex beads (Sigma). All other chemicals and reagents were from Sigma-Aldrich. Plasmid and constructs The mouse PI3Kγ cDNA was obtained from the Facility for Life Science Automation at the Institute for Molecular Bioscience. GST-PI3Kγ-FL and His-PI3Kγ-FL were expressed in Sf9 insect cells using baculovirus expression vector systems according to the manufacturer’s instructions (Invitrogen). Rab8a was subcloned into pEGFP-C1, pm-Cherry-C1 and ptd-Tomato-C1 that had been generated from pCMV-tdTomato (Clontech). The pEGFP-Rab8aCAAX domain (Rab8a tail) was generated by PCR to contain the last 29 amino acids of the Rab8a C terminus with a modification of the CAAX motif to CMIV to allow for prenylation of the fusion protein [53] , [54] . Rab8a was also subcloned into pGEX6P-1 and expressed in E. coli [55] . Phosphoinositide probes and pEGFP-C1-Akt-PH were kindly provided by Frederic Meunier, and the lentiviral vector PLL5.0 was obtained from Alpha Yap (both of The University of Queensland, QLD, Australia). Mal–Cerulean and TLR4-Citrine plasmids were gifts from Nicholas J. Gay, University of Cambridge, UK. Expression and purification of recombinant proteins Recombinant GST-tagged proteins were produced in an E. coli BL21(DE3) strain transformed with the plasmid DNA of interest. Expression of the recombinant protein was induced with the addition of 0.5 mM IPTG for 18 h at 25 °C with shaking. The bacterial cells were then pelleted by centrifugation at 5,000 g . The pellets were resuspended in ice-cold lysis buffer (Tris pH 7.4, 300 mM NaCl, 1 mM EDTA, cOmplete EDTA-free protease inhibitor cocktail tablet (Roche Applied Science), 1 mM DTT and 1 mM PMSF). The bacterial lysates were lysed using a Constant Systems cell disruptor according to the manufacturer’s instructions (Thermo Scientific, Australia) and then cleared by centrifugation at 48,254 g at 4 °C. The recombinant proteins were affinity purified by incubating the cleared lysate with Glutathione Sepharose (GE Healthcare Life Science, Australia) for 1 h at 4 °C. The beads were washed extensively with 1 M NaCl in 20 mM Tris pH 7.4. GST-fusion proteins on the beads were stored at −20 °C in 20 mM Tris pH 7.4 containing 20% glycerol. Mouse model Knockout of the p110γ subunit in PI3Kγ −/− mice (pik3cg2/2) on a C57BL/6 background has been previously described [28] . Age (16–20 weeks) and sex-matched C57BL/6 mice were used as controls. Mice were housed and used for experiments in accordance with approved animal ethics protocols at AMREP (Alfred Medical Research and Education Precinct) AEC, Alfred Hospital Melbourne, Victoria. (E/1089/2011/M). Experiments utilized samples or cells from three or more mice per group per time point to generate statistical significance. Animals within groups were randomized for treatments. Primary BMMs were obtained by ex vivo differentiation of bone marrow cells collected from mouse femurs or tibias. Cells were differentiated for 7 days in complete RPMI medium supplemented with 20 U ml −1 penicillin, 20 μg ml −1 streptomycin and 100 ng ml −1 purified recombinant macrophage colony-stimulating factor-1 (refs 56 , 57 ). Cell culture and siRNA The mouse RAW 264.7 macrophage cell line was sourced from ATCC. PI3Kγ was silenced using Stealth siRNA primer sets from Life Technologies, Australia (catalogue number 1320003). RAW 264.7 macrophages were cultured in RPMI 1640 medium (Lonza) supplemented with 10% heat-inactivated FCS (Thermo Trace) and 2 mM L-glutamine (Invitrogen) in humidified 5% CO 2 at 37 °C (ref. 58 ). Cells were screened monthly for mycoplasmal contamination. For transient expression of cDNA, cells at 50% confluence were transfected using Lipofectamine 2000 (Invitrogen) according to the manufacturer’s instructions. Cells were typically used for experiments 18 h after transfection. Non-targeting siRNA was used as a control. For Rab8a depletion, an 18 nucleotide shRNA was designed and cloned into the lentivirus expression vector LentiLox pLL5.0 (refs 59 , 60 , 61 ), using forward primer 5′-tGCCTTCAACTCCAC ATTCAttcaagagaTGAATGTGGAGTTGAAGGCttttttg-3′, and reverse primer 5′-TCGACAAAAAAGCCTTCAACTCCACATTCATCTCTTGAATGAATGTGGATTGAAGGCA-3′. The shRNA was cloned downstream of the U6 promoter (HpaI and XhoI) into a lentivirus expression vector pLL5.0 (backbone pLL3.7) carrying a soluble mCherry gene as a fluorescent reporter. The pLL5.0 shRNA and packaging vectors were transfected into HEK-293T cells by Lipofectamine 2000 precipitation. Virus-like particles were collected from the supernatant 48–72 h after transfection, and virus was concentrated using polyethylene glycol 6000 (ref. 62) [62] . Aliquots of virus were subsequently used for titration or stored at −80 °C. Titres were determined by infecting HEK-293T cells with serial dilutions of concentrated lentivirus. RAW 264.7 macrophages were infected with lentiviral particles at a multiplicity of infection of 10 per cell. Cells were incubated at 37 °C with lentivirus in RPMI complete medium and collected 48 h post infection. Single-cell suspensions were sorted by flow cytometry according to moderate to high levels of reporter gene expression. Fixed cell ruffle quantification and analysis RAW 264.7 macrophages were grown on coverslips overnight at a low confluency. Cells were either treated with exogenous LPS 100 ng ml −1 (stimulated) or not treated (unstimulated) for 30 min before fixation. Cytoskeletal F-actin was labelled with Alexa Fluor 488 phalloidin (Life Technologies) for 60 min; in addition, nuclei were labelled with 4',6-diamidino-2-phenylindole (DAPI) concurrently. Three-dimensional z -stacks were acquired using a DeltaVision devolution microscope (GE Healthcare) and were analysed using Fiji image software. The mid-point of cellular nuclei (DAPI) was selected and labelled as the new base slice. Slices from the mid-point until the top of the cell were flattened using maximum projection. Background subtraction and median filters were applied to the flattened image for smoothing purposes for further analysis. The image was then duplicated, whereby a threshold mask was constructed (equally for all images) and all regions collected from the phalloidin threshold image were selected as the region of interest (ROI). The fluorescence intensity for the generated ROI in the phalloidin channel was then measured and quantified using GraphPad Prism. Phagocytic assay and procedures Wild-type and PI3Kγ −/− BMMs ( n =3 each) were grown on coverslips before phagocytosis experiments. Latex beads (3 μm diameter) from Sigma-Aldrich (LB30-2ML) were diluted 1 × 10 −1 in dH2O and washed with phosphate-buffered saline (PBS) three times by centrifugation. Beads were resuspended in 2 μg ml −1 human immunoglobulin G (IgG) (Invitrogen, 02-7102) in PBS. IgG was left to bind by passive adsorption for 2 h at room temperature on a rotating mixer. The suspension was then washed three times and resuspended in PBS and sodium azide (0.2%). For phagocytosis, 1 μl of this suspension was added to macrophages on coverslips in 1 ml of cold complete RPMI medium, and spun onto the cells at 1,00 g for 2 min at 4 °C. Cells are then transferred back to 37 °C for 5–20 min. Cells were fixed in 4% paraformaldehyde for 30 min and then permeabilized, if required, with 0.1% Triton X-100/PBS for 5 min. Washing, blocking and antibody incubation steps were done using blocking buffer (0.5% BSA/PBS). Human IgG on beads was detected using Cy3 goat anti-human antibody (1:200, Jackson Labs 109-165-003). Cells were labelled with Alexa350/488 phalloidin (1:50/1:500, Molecular Probes, 22281,12379), to outline cells and show actin-enrichment at sites of phagocytosis. Coverslips were mounted in Prolong Gold (Invitrogen, P10144) for imaging. Olympus BX-51 upright microscope fitted with an Olympus DP-71 12Mp Colour Camera. Images were captured using a × 40/1.35 U Apo Oil lens with the Olympus DP controller version 2.1 capture software at an image size of 2040 × 1536 pixels. Each bead was classified as either phagocytosed (Cy3<5%), in-between (5%<Cy3<95%) or attached (Cy3 >95%) for comparison between groups [63] . ( n >200 beads per animal). TLR4 internalization assay Wild-type and PI3Kγ −/− BMMs ( n =3 each) were grown on non-adherent tissue culture plates. In FACS tubes, 0.5 × 10 6 cells ml −1 for each animal in triplicate were treated with or without LPS (100 ng ml −1 ) for indicated times at 37 °C before being placed on ice to halt all internalization. Cells were washed twice with ice-cold FACS buffer (PBS, 1% FCS, 5 mM EDTA) and blocked with 24G2 for 20 min on ice. Cell surface TLR4 was stained with biotinylated anti-TLR4 (clone SA15-21 Biolegend 145402) at 0.5 μg ml −1 . Cells were washed three times in FACS buffer before labelling with Streptavidin–APC (Biolegend 405207) at 0.5 μg ml −1 . Cells were washed extensively in FACS buffer at 4 °C before acquisition on a Canto II cytometer (Becton Dickinson). Cellular profiles were analysed using FlowJo software (TreeStar). The percentage internalization=(MFI X −MFI TLR4−/− )/(MFI WT untreated −MFI TLR4−/− ) × 100 for each data point. Transferrin uptake assay Wild-type and PI3Kγ −/− BMMs ( n =3 each) grown on coverslips were serum starved for 30 min and treated with Alexa Fluor 546-labelled mouse transferrin (Life Technologies) for 10 min at 37 °C. Cells were then washed and chased for 20 min at 37 °C in complete medium to allow trafficking of transferrin from early endosomes to recycling endosomes. Flattened three-dimensional images were captured for each treatment using identical conditions. The background intensity ROI was selected from a region not containing cells. Background intensity was removed from the entire field of view before individual cells were selected, and total cell transferrin intensity was then measured for analysis ( n >30 cells per animal). Dextran uptake assay RAW 264.7 macrophages were incubated with or without LPS pre-priming for 30 min. Alexa Fluor 488-conjugated dextran (10,000 MW) was added to the cells at a final concentration of 50 μg ml −1 in complete medium and left on cells for 10 min. Macropinocytosis was stopped by washing cells in 4 °C PBS before exchanging for 4 °C complete medium. Cells were kept on ice until imaging live using the Personal DeltaVision deconvolution microscope. Macropinocytosis was then analysed using ImageJ software. Cells were segmented using WGA as a cell mask. Macropinosomes were segmented and filtered by size >0.2 μm. Final segmentation of individual macropinosomes was performed manually before counting and size measurements were taken in an automated fashion. Ruffle enrichment analysis Recruitment analysis was performed by comparing the fluorescence intensity of a transfected protein at multiple locations in a given cell. The peak fluorescence intensity of each channel across an ROI line was divided by the fluorescent intensity of WGA as a measure of total membrane. The mean fluorescence of each channel/WGA at the filopodia was set to 1 and the measurements in ruffles compared with identify recruitment of tdTomato-Rab8a and GFP-Akt-PH. By standardizing all measurements to the WGA intensity at the filopodia, measurements among cells could be compared even though the total intensity per cell was not equal. Microscopy For live cell experiments, RAW 264.7 macrophages were cultured on glass-bottom 35-mm dishes (MatTek). Live and fixed cell imaging were additionally performed using a Personal DeltaVision Olympus IX71 inverted wide-field deconvolution microscope equipped with Olympus U-Apochromat 40 × /1.35 oil DIC, Plan-Apochromat 60 × /1.42 oil DIC and UPLS-Apochromat 100 × /1.40 oil DIC, and a 120 W xenon arc lamp. Images were captured using a Roper Coolsnap HQ2 monochrome camera. Live cell three-dimensional z -stack imaging for ruffle analysis using temporal colour coding was acquired using the Zeiss Axiovert 200 Yokogawa spinning disk confocal microscope. Each stack was acquired every 30 s and full stacks represented as sum-intensity projections. Temporal colour coding of each slice was performed using ImageJ and the spectrum lookup table. Immunofluorescence staining is described in ‘phagocytic assay and procedures’ [63] , [64] . Scanning electron microscopy RAW 264.7 macrophage cells were incubated with human IgG-opsonized latex beads (3 μm, Sigma-Aldrich) for 30 min and fixed with 2.5% glutaraldehyde in sodium cacodylate buffer, post-fixed in 2% osmium tetroxide, dehydrated through ethanol, and dried using HMDS (Sigma-Aldrich). Coverslips were coated in platinum and viewed on a JEOL JSM-6300F scanning electron microscope. Immunoblot For immunoblot analysis [65] , cells were lysed in lysis buffer (20 mM HEPES pH 7.4, 100 mM NaCl, 1% NP-40 (Sigma) with addition of 1 mM PMSF, 1 mM DTT, cOmplete protease inhibitors (Roche Applied Science) and phospho-Stop tablets (Roche Applied Science). The proteins were transferred to a polyvinylidene difluoride membrane (BioTrace, NZ), blocked with 5% skim milk in PBS-0.1% Tween-20 buffer (TBS-T) and incubated overnight at 4 °C with primary antibodies. After washing of the membrane, a secondary antibody was incubated for 1 hour. The membrane was developed with a chemiluminescence reagent (ECL, Detection Reagents, Thermo Scientific) according to the manufacturer’s instructions. Quantitative real-time PCR and enzyme-linked immunosorbent assay Total RNA was prepared using RNeasy mini-kits (Qiagen, Valencia, CA) and cDNA reverse transcribed using 1 μg of total RNA and Superscript III reverse transcriptase (Invitrogen, Carlsbad, CA). Gene expression was quantitated using SYBR Green PCR master mix (Applied Biosystems) [66] , using an ABI Prism 7000 sequence detection system (Applied Biosystems, Foster City, CA). All primers used in this study are listed in Supplementary Table 2 . Data are presented as relative change compared with control cells ( n =3) and represents the average±s.e.m. Rab8a GTP loading for GST pull-down and mass spectrometry analysis GTP-loaded GST-Rab8a sepharose beads were incubated with LPS-activated cell lysate for 1 h at 4 °C with agitation. MicroSpin columns (#27– 3565–01; GE Healthcare) were used for all of the pull-downs. Beads were washed with ice-cold wash buffer (50 mM Tris, 150 mM NaCl, 1% NP-40, 1 mM PMSF, 1 mM DTT, pH 7.4). Elution was achieved conventionally by boiling in 3 × SDS–PAGE sample buffer for 5 min (ref 67 ). LC MS/MS was performed at the IMB Mass Spectrometry Facility, The University of Queensland. LPS-stimulated RAW 264.7 macrophage extracts were lysed in ice-cold lysis buffer (20 mM HEPES pH 7.4, 150 mM NaCl, 1% NP-40 (Sigma), 1 mM PMSF, 1 mM DTT, cOmplete protease inhibitors (Roche Applied Science), and PhosStop tablet (Roche Applied Science). The lysate was centrifuged at 75,600 g for 15 min at 4 °C. The supernatant was pre-cleared by the addition of GSH-Sepharose beads for 1 h, pelleted at 50 g for 5 min at 4 °C, and the supernatant collected. Various GST-tagged recombinant proteins were then incubated with an equal amount of tissue lysate at 4 °C for 1 h. Beads were washed extensively with ice-cold 20 mM Tris pH 7.4 containing 150 mM NaCl, 1 mM DTT, and 1 mM PMSF, eluted in 2 × SDS–PAGE sample buffer, resolved on 10% SDS–PAGE gels, and stained with Coomassie blue G250. GTP loading of Rab8 was performed by nucleotide exchange as described earlier [68] . Samples were analysed by LC MS/MS on a Shimadzu Prominence Nano HPLC (Japan) coupled to a Triple TOF 5600 mass spectrometer (ABSCIEX, Canada) equipped with a nano electrospray ion source. Six microliters of each extract was injected onto a 50 mm × 300 μm C18 trap column (Agilent Technologies, Australia) at 30 μl min −1 . The samples were de-salted on the trap column for 5 min using 0.1% formic acid at 30 μl min −1 . The trap column was then placed in-line with the analytical nano HPLC column, a 150 mm × 75 μm 300SBC18, 3.5 μm (Agilent Technologies, Australia) for mass spectrometry analysis. Linear gradients of 1–40% solvent B over 35 min at 300 nl min −1 flow rate, followed by a steeper gradient from 40 to 80% solvent B in 5 min were used for peptide elution. Solvent B was held at 80% for 5 min for washing the column, and then returned to 1% solvent B for equilibration before the next sample injection. Solvent A consisted of 0.1% formic acid and solvent B contained 90/10 acetonitrile/0.1% formic acid. The ion spray voltage was set to 2400 V, declustering potential (DP) 100 V, curtain gas flow 25, nebuliser gas 1 (GS1) 12, and interface heater at 150 °C. The mass spectrometer acquired 500 ms full scan TOF-MS data followed by 20 by 50 ms full scan product ion data in an information dependent acquisition (IDA) mode. Full scan TOF-MS data were acquired over the mass range 350–1400 and for product ion ms/ms 80–1400. Ions observed in the TOF-MS scan exceeding a threshold of 100 counts and a charge state of +2 to +5 were set to trigger the acquisition of product ion, ms/ms spectra of the resultant 20 most intense ions. The data were acquired and processed using Analyst TF 1.6.1 software (ABSCIEX, Canada). Proteins were identified by database searching usingProteinPilot v4.5 (ABSCIEX, Canada) against the UniProt_Sprot_20130205 database (~106,000 entries of all species searched, FDR of 1%). Search parameters were defined as a thorough search using trypsin digestion, iodoacetamide cysteine alkylation and all entries in the database. Proteins were considered identified if there was at least one peptide identified with 99% confidence. Image analysis software All images were analyzed using either ImageJ (version 1.43; National Institutes of Health, Maryland, USA) or Imaris (version 7.3.6, Bitplane Scientific Software). Adobe Photoshop CS6 was used to crop regions of interest or to extract single channels. Statistics If not stated otherwise, data are presented as arithmetic means±s.e.m. For direct comparison of one experimental variation, Student’s t -test was used for data with normal distribution (assessed by Shapiro–Wilk test). Post-test analysis of one-way analysis of variance was corrected for multiple comparisons by Dunett’s method and corrected for multiple comparisons in two-way analysis of variance using Sidak’s method. All analysed experiments used biological replicates to compute statistical significance. In all statistical analysis, a P- value<0.05 was considered statistically significant. Statistics were calculated using GraphPad Prism version 7.0 (GraphPad Software, San Diego, CA). How to cite this article : Luo, L. et al. Rab8a interacts directly with PI3Kγ to modulate TLR4-driven PI3K and mTOR signalling. Nat. Commun. 5:4407 doi: 10.1038/ncomms5407 (2014).